Probing backbone hydrogen bonding in PDZ/ligand interactions by protein amide-to-ester mutations PDZ domains are scaffolding modules in protein–protein interactions that mediate numerous physiological functions by interacting canonically with the C-terminus or non-canonically with an internal motif of protein ligands. A conserved carboxylate-binding site in the PDZ domain facilitates binding via backbone hydrogen bonds; however, little is known about the role of these hydrogen bonds due to experimental challenges with backbone mutations. Here we address this interaction by generating semisynthetic PDZ domains containing backbone amide-to-ester mutations and evaluating the importance of individual hydrogen bonds for ligand binding. We observe substantial and differential effects upon amide-to-ester mutation in PDZ2 of postsynaptic density protein 95 and other PDZ domains, suggesting that hydrogen bonding at the carboxylate-binding site contributes to both affinity and selectivity. In particular, the hydrogen-bonding pattern is surprisingly different between the non-canonical and canonical interaction. Our data provide a detailed understanding of the role of hydrogen bonds in protein–protein interactions. Protein–protein interactions (PPIs) are vital for almost all cellular and biochemical processes and are attractive as novel and promising drug targets, in which inhibitors of PPIs comprise exciting therapeutic prospects [1] , [2] . The PDZ (postsynaptic density-95, Drosophila discs-large, zona occludens 1) protein domain family is one of the largest classes of PPI domains in the human genome. PDZ domains increase the specificity and efficiency of intracellular communication networks downstream of receptor activation by facilitating several PPIs [3] , [4] . The human genome contains an estimated 256 PDZ domains in 142 different proteins [5] . PDZ domains are often found in multidomain scaffold and anchoring proteins involved in trafficking, recruiting and assembling of intracellular enzymes and membrane receptors into signalling-transduction complexes [6] , [7] . Many PDZ domains are putative drug targets [8] , [9] , [10] , such as PDZ domains of PSD-95, in which inhibitors are pursued for treatment of ischemia and neuropathic pain [11] , [12] , [13] , [14] . In addition to their physiological and therapeutic relevance, PDZ domains are frequently used as a model system to explore fundamental aspects of protein folding [15] , ligand/protein interactions [10] , [16] and allostery [16] , [17] . PDZ domains are made up of five to six antiparallel β-strands (β1–β6) and two to three α-helices (α1–α3). In the canonical binding mode, the C-terminal of the interacting protein binds as an additional antiparallel β-strand within a groove between the β2 strand and α2 helix ( Fig. 1a ) [18] , [19] . The C-terminal carboxylate of the peptide ligand is anchored at the carboxylate-binding site, which is a characteristic loop between β1 and β2 strands containing a highly conserved four amino-acid sequence motif X 1 -Φ 1 -G-Φ 2 (X: any amino acid; Φ: hydrophobic residue; G: Gly). The importance of the amino-acid side chains in the C-terminal peptide ligand for interaction with PDZ domains has been thoroughly studied, providing a generally accepted binding mode. The last four residues (P 0 –P -3 ) of the peptide ligand are major determinants for binding, and side chains of residues P 0 and P -2 are particularly important for ligand affinity and selectivity [20] , [21] , [22] . 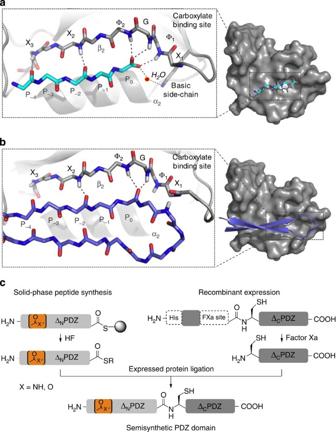Figure 1: Canonical and non-canonical interactions of the PDZ domains. (a) X-ray crystal structure of C-terminal peptide ligand (cyan) in complex with a PDZ domain (grey) demonstrating the canonical binding mode (PDB ID 1BE9). Three H-bonds are formed at the carboxylate-binding site (X1Φ1GΦ2) from the PDZ domain backbone amide NH of Φ1, G and Φ2to the C-terminus of the peptide ligand. The side-chain of a conserved basic amino acid coordinates a water molecule (orange) which donates an additional H-bond to the carboxylate. For certain canonical PDZ/ligand interactions, functional studies45,46have shown that the backbone amides NHs of X2and X3(and carbonyls of Φsand X2, not shown) in the PDZ domain may participate in H-bond donation to the amide carbonyls in P-1,-2and P-3,-4, respectively, of the C-terminal ligand. The X-ray crystal structure from the first co-crystallized PDZ/ligand complex18has been used for illustrating the probed H-bond patterns. (b) X-ray crystal structure of the interaction between internal β-finger ligand (purple) and PDZ domain (grey) demonstrating the non-canonical binding mode (PDB ID 1QAV). The β-finger ligand aligns with the β2 strand of the PDZ domain forming an extended antiparallel β sheet forming two H-bonds from the backbone amide NH of G and Φ2in the carboxylate-binding site to the β-finger ligand along with one H-bond from backbone amides NH of X2. (c) Schematic representation of the strategy for the semisynthesis of the PDZ domains. The N-terminal fragment is prepared by SPPS, which allows introduction of backbone mutations. The synthesized thioester peptide is cleaved from the resin using anhydrous HF. The C-terminal fragment is recombinantly expressed and enzymatically treated by FXa enzyme, which removes the polyhistidine tag (His) and generates a terminal Cys. The two fragments are subsequently ligated yielding the full-length PDZ domain. Figure 1: Canonical and non-canonical interactions of the PDZ domains. ( a ) X-ray crystal structure of C-terminal peptide ligand (cyan) in complex with a PDZ domain (grey) demonstrating the canonical binding mode (PDB ID 1BE9). Three H-bonds are formed at the carboxylate-binding site (X 1 Φ 1 GΦ 2 ) from the PDZ domain backbone amide NH of Φ 1 , G and Φ 2 to the C-terminus of the peptide ligand. The side-chain of a conserved basic amino acid coordinates a water molecule (orange) which donates an additional H-bond to the carboxylate. For certain canonical PDZ/ligand interactions, functional studies [45] , [46] have shown that the backbone amides NHs of X 2 and X 3 (and carbonyls of Φ s and X 2 , not shown) in the PDZ domain may participate in H-bond donation to the amide carbonyls in P -1,-2 and P -3,-4 , respectively, of the C-terminal ligand. The X-ray crystal structure from the first co-crystallized PDZ/ligand complex [18] has been used for illustrating the probed H-bond patterns. ( b ) X-ray crystal structure of the interaction between internal β-finger ligand (purple) and PDZ domain (grey) demonstrating the non-canonical binding mode (PDB ID 1QAV). The β-finger ligand aligns with the β2 strand of the PDZ domain forming an extended antiparallel β sheet forming two H-bonds from the backbone amide NH of G and Φ 2 in the carboxylate-binding site to the β-finger ligand along with one H-bond from backbone amides NH of X 2 . ( c ) Schematic representation of the strategy for the semisynthesis of the PDZ domains. The N-terminal fragment is prepared by SPPS, which allows introduction of backbone mutations. The synthesized thioester peptide is cleaved from the resin using anhydrous HF. The C-terminal fragment is recombinantly expressed and enzymatically treated by FXa enzyme, which removes the polyhistidine tag (His) and generates a terminal Cys. The two fragments are subsequently ligated yielding the full-length PDZ domain. Full size image It is well established that the C-terminal carboxylate interaction with the carboxylate-binding site is preserved and fundamental to all PDZ domains, yet surprisingly little is known about the functional and molecular details of this interaction. Structural studies show that the C-terminal carboxylate forms three hydrogen bonds (H-bonds) with backbone amides in the carboxylate-binding site along with a water-mediated H-bond coordinated by a conserved basic residue (Arg/Lys) [18] , [23] , [24] . Mutation of this residue has a limited effect on ligand binding [25] , [26] , [27] , suggesting an essential role of the backbone amides in the carboxylate-binding site. Some PDZ domains also recognize internal peptide motifs lacking a free carboxylate C-terminus, such as a β-finger motif from neuronal nitric oxide synthase (nNOS) that interacts with PDZ domains from PSD-95, syntrophin and ZO-1 (refs 28 , 29 , 30 ), and which has been exploited as scaffold for developing inhibitors of PDZ domains [31] . The backbone of the β-finger also aligns as an antiparallel β sheet to the β2 strand of the PDZ domain ( Fig. 1b ) and supposedly share the same H-bond pattern as the C-terminal peptide ligand [28] . Since protein backbone interactions in general cannot be addressed by conventional mutational analysis, alternative strategies have been pursued [32] , [33] . Here we employ expressed protein ligation (EPL) [34] , [35] to generate PDZ domains with amide-to-ester (A-to-E) mutations [36] to dissect canonical and non-canonical interactions in prototypical PDZ domains. We observe dramatic effects on ligand binding upon A-to-E mutations and demonstrate major differences between the two binding modes. Our results provide new insight into the molecular details of ligand/PDZ domain interactions, which are pertinent for the fundamental understanding of PDZ domains, including their widespread use as model systems and in the development of novel efficient inhibitors of PDZ domains. Semisynthesis of PDZ domains We selected the PSD-95-PDZ2 domain as a target for our initial development of a semisynthetic strategy, as PSD-95 is a prototypical PDZ domain protein [37] , [38] , in which the PDZ2 domain of PSD-95 (PSD-95-PDZ2) binds both linear C-terminal peptides and a β-finger ligand. In PSD-95-PDZ2, the carboxylate-binding site (L170, G171 and F172), as well as other possible backbone H-bond interactions of the β2 strand (I174 and G176) are located in the N-terminal region of the PDZ domain ( Supplementary Fig. 1 ). Hence, to introduce backbone mutations in this region by EPL, we envisioned a strategy in which a modified N-terminal ester-containing peptide thioester (Δ N PDZ) and a C-terminal protein fragment with an N-terminal Cys (Δ C PDZ) are prepared by solid-phase peptide synthesis (SPPS) and recombinant expression, respectively. The two fragments can then undergo a chemoselective ligation generating the full-length PDZ domain ( Fig. 1c ). A Cys scanning mutagenesis of PSD-95-PDZ2 identified V178 as a ligation site, since the V178C mutant maintained wild-type (WT) ligand-binding affinity ( Supplementary Figs 1 and 2 ). Thus, A-to-E mutations of all planned positions can be achieved by ligation of a synthetic 23 amino-acid peptide thioester containing A-to-E mutations and a recombinantly expressed C-terminal 72 amino-acid protein. As an initial test of our EPL approach, we prepared the WT semisynthetic (WT SS ) PSD-95-PDZ2 to ensure that the strategy could yield sufficient amounts of protein with native fold and intact ligand binding. The PSD-95-PDZ2 N-terminal peptide thioester fragment ( 1 , Δ N PDZ2) was prepared by Boc/ t Bu SPPS ( Fig. 2a,b ). The C-terminal protein fragment ( 2 , Δ C PDZ2) was obtained by expression in Escherichia coli of PSD-95-PDZ2, with a polyhistidine tag in the N-terminal and a Factor Xa (FXa) cleavage site in front of position V178C. The purified protein was subjected to FXa cleavage and the desired protein 2 was obtained in good yield and purity ( Fig. 2c,d ). The ligation of peptide 1 (Δ N PDZ2) and protein 2 (Δ C PDZ2) generated full-length PSD-95-PDZ2 3 ( Fig. 2e,f ), which was purified and refolded by dialysis to provide WT SS PSD-95-PDZ2 4 . The secondary structure and ligand binding of 4 was examined by circular dichroism (CD) ( Supplementary Fig. 3 ) and in a saturation binding fluorescence polarization (FP) assay using a fluorescent-labelled GluN2B peptide (Cy5-CSGYEKLSSIESDV) [39] , respectively ( Fig. 3a,b ). These results show that secondary structures and ligand affinities of WT and WT SS PSD-95-PDZ2 are similar, demonstrating that the devised EPL strategy allows expedient preparation of semisynthetic PSD-95-PDZ2 protein with properties identical to those of the recombinantly expressed protein. 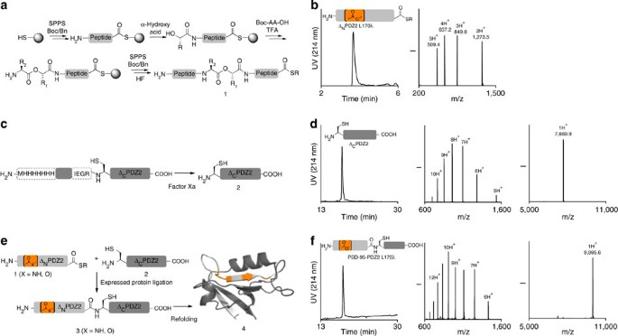Figure 2: Semisynthesis of backbone-modified PSD-95-PDZ2. (a) Synthesis of the N-terminal peptide fragment of PSD-95-PDZ2. The peptide thioester was prepared using Boc/Bn-based SPPS on a preloaded resin containing a free thiol. A backbone ester was introduced by coupling of an α-hydroxy acid followed by a Boc-protected amino acid. The deprotections were performed using TFA and the peptide was cleaved with HF generating the N-terminal fragment ΔNPDZ2. (b) LC-MS characterization of ester-containing thioester peptide fragment ΔNPDZ2 L170λ. Chromatogram at UV λ214 nmand ESI mass spectra (1H+observed mass 2,546.9 Da, calculated 2,547.3 Da). (c) Recombinant expression of the C-terminal fragment of PSD-95-PDZ2. A fusion protein containing ΔCPDZ2 along with an N-terminal poly-histidine tag (MHHHHHHH) and a Factor Xa recognition site (IEGR) was overexpressed inE. coliand subsequently purified. The protein was subjected to enzymatic digestion with Factor Xa, generating fragment2(ΔCPDZ2). (d) Characterization of ΔCPDZ2. RP-HPLC chromatogram (UV λ214 nm), ESI mass spectra and deconvoluted peak (1H+observed mass 7,669.9 Da, calculated 7,669.2 Da). (e) Ligation and refolding of semisynthetic PSD-95-PDZ2. The thioester peptide fragment1(ΔNPDZ2) and the expressed fragment2(ΔCPDZ2) were ligated generating full-length semisynthetic PSD-95-PDZ23. The denatured protein was subsequently refolded by dialysis generating4. (f) Characterization of the ligation product PSD-95-PDZ2 L170λ. RP-HPLC chromatogram (UV λ214 nm), ESI mass spectra and deconvoluted peak (1H+observed mass 9,995.6 Da, calculated 9,996.0 Da). Figure 2: Semisynthesis of backbone-modified PSD-95-PDZ2. ( a ) Synthesis of the N-terminal peptide fragment of PSD-95-PDZ2. The peptide thioester was prepared using Boc/Bn-based SPPS on a preloaded resin containing a free thiol. A backbone ester was introduced by coupling of an α-hydroxy acid followed by a Boc-protected amino acid. The deprotections were performed using TFA and the peptide was cleaved with HF generating the N-terminal fragment Δ N PDZ2. ( b ) LC-MS characterization of ester-containing thioester peptide fragment Δ N PDZ2 L170λ. Chromatogram at UV λ 214 nm and ESI mass spectra (1H + observed mass 2,546.9 Da, calculated 2,547.3 Da). ( c ) Recombinant expression of the C-terminal fragment of PSD-95-PDZ2. A fusion protein containing Δ C PDZ2 along with an N-terminal poly-histidine tag (MHHHHHHH) and a Factor Xa recognition site (IEGR) was overexpressed in E. coli and subsequently purified. The protein was subjected to enzymatic digestion with Factor Xa, generating fragment 2 (Δ C PDZ2). ( d ) Characterization of Δ C PDZ2. RP-HPLC chromatogram (UV λ 214 nm ), ESI mass spectra and deconvoluted peak (1H + observed mass 7,669.9 Da, calculated 7,669.2 Da). ( e ) Ligation and refolding of semisynthetic PSD-95-PDZ2. The thioester peptide fragment 1 (Δ N PDZ2) and the expressed fragment 2 (Δ C PDZ2) were ligated generating full-length semisynthetic PSD-95-PDZ2 3 . The denatured protein was subsequently refolded by dialysis generating 4 . ( f ) Characterization of the ligation product PSD-95-PDZ2 L170λ. RP-HPLC chromatogram (UV λ 214 nm ), ESI mass spectra and deconvoluted peak (1H + observed mass 9,995.6 Da, calculated 9,996.0 Da). 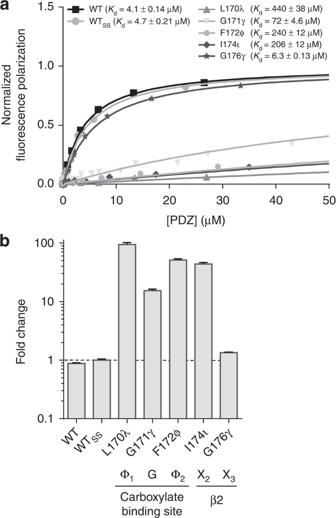Figure 3: The canonical interaction of PSD-95-PDZ2 domains with A-to-E mutations. (a) Saturation curves from FP assay. Increasing amounts of PSD-95-PDZ2 was titrated against a Cy5-labelled GluN2B C-terminal peptide ligand (Cy5-CYEKLSSIESDV). TheKdvalues were determined for the controls (WT, WTSS) and five different A-to-E mutants having backbone mutations introduced in either the carboxylate-binding site (L170λ, G171γ, F172ϕ) or in the β2 strand (I174τ, G176γ). The affinity constants are reported asKd±s.e.m. (b) The fold change in affinity towards the GluN2B C-terminal peptide ligand reported relative to the control WTSS(Kd(mutant)/Kd(WTSS)±s.e.m). Full size image Figure 3: The canonical interaction of PSD-95-PDZ2 domains with A-to-E mutations. ( a ) Saturation curves from FP assay. Increasing amounts of PSD-95-PDZ2 was titrated against a Cy5-labelled GluN2B C-terminal peptide ligand (Cy5-CYEKLSSIESDV). The K d values were determined for the controls (WT, WT SS ) and five different A-to-E mutants having backbone mutations introduced in either the carboxylate-binding site (L170λ, G171γ, F172ϕ) or in the β2 strand (I174τ, G176γ). The affinity constants are reported as K d ±s.e.m. ( b ) The fold change in affinity towards the GluN2B C-terminal peptide ligand reported relative to the control WT SS ( K d (mutant)/ K d (WT SS )±s.e.m). Full size image We then proceeded to introduce A-to-E mutations in PSD-95-PDZ2 using the EPL strategy. Specifically, we introduced mutations in the carboxylate-binding site (L170λ, G171γ and F172ϕ) and two sites in the β2 strand (L170λ and G176γ). The corresponding five ester-containing peptide thioesters were prepared by incorporation of an α-hydroxy acid [40] , [41] and were used in subsequent ligation reactions with protein fragment 2 (Δ C PDZ2), and upon dialysis the five PSD-95-PDZ2 proteins containing A-to-E mutations were obtained. CD spectra suggested that all five semisynthetic ester-containing proteins obtained the same overall fold as WT PSD-95-PDZ2 ( Supplementary Fig. 3 ), which was expected as PDZ domains generally refold very well [42] , and previous X-ray crystal structures have shown that A-to-E mutations can be introduced without perturbing the overall or backbone structure [43] , [44] . Thus, an efficient procedure for the semisynthesis of structurally intact PDZ domains was developed and used to introduce backbone A-to-E mutations. Backbone H-bonds in the PSD-95-PDZ2/GluN2B interaction The ligand-binding properties of WT PSD-95-PDZ2 and the five A-to-E mutants were tested in the FP assay ( Fig. 3a ). Comparison of the K d values for binding of the GluN2B peptide ligand to WT SS and the L170λ, G171γ and F172ϕ mutants revealed remarkable effects of removal of the H-bond donor capacity for all three backbone positions in the carboxylate-binding site ( Fig. 3b ). Specifically, each individual A-to-E mutation leads to dramatic decreases in affinity of the ligand; producing 94-, 15- and 51-fold loss of affinity for L170λ, G171γ and F172ϕ, respectively, compared with WT SS . Introduction of a backbone ester at I174 and G176 in the β2 strand that have been proposed to be important contributors to binding for other PDZ/ligand interactions [45] , [46] showed that only the I174τ mutation affected ligand binding, producing a 44-fold loss in affinity, whereas ligand affinity was not affected by the G176γ mutation ( Fig. 3b ), in agreement with structural data. We then examined the kinetic properties of the interaction using the stopped-flow technique by rapidly mixing A-to-E-mutated PSD-95-PDZ2 domains with a fluorescent C-terminal peptide ligand (dansyl-SIESDV) ( Supplementary Table 1 ). The experiments confirmed the notable effects of the A-to-E mutations on the affinity, and the lower affinities from the mutations in positions L170, F172 and I174 led to increased off-rate constants ( k off ) such that resulting observed rate constants were too fast for the stopped-flow instrument. Kinetic binding traces from changes in fluorescence were obtained for PSD-95-PDZ2 WT SS as well as the G171γ and G176γ mutants showing that the kinetics for WT SS and G176γ was very similar, confirming that the backbone amide of G176 is not involved in binding the ligand. Interestingly, the G171γ mutant showed an increase in the association rate constant k on (15±3 versus 3.2±0.4 μM −1 s −1 ; Supplementary Table 1 ), suggesting that the backbone amide NH forms an unfavourable interaction during the rate-limiting step of the association of the ligand. Together, these results demonstrate that backbone interactions in PSD-95-PDZ2 are critical for binding of a native peptide ligand and provide a quantitative measure of the relative contribution of individual backbone interactions for ligand affinity (L170>F172>I174>G171>>G176). Backbone H-bonds in four PDZ domains PDZ domains have generally been grouped into three classes (I, II and III) depending on the identity of the amino acids in P 0 and P -2 of the C-terminal peptide ligand, although an unambiguous classification still remains a challenge [21] , [22] . PSD-95-PDZ2 is a class I PDZ domain as it binds the general C-terminal sequence S/T-X-V/L [20] . To address the importance of the backbone amide NH interactions across PDZ domain classes, four PDZ domains representing classes II and III were selected for similar analysis. We included PDZ domains from membrane protein palmitoylated 7 (MPP7-PDZ) and regulator of G protein signalling 3 (RGS3-PDZ), as representatives for class II (Φ-X-Φ), as well as from nNOS (nNOS-PDZ) and zonula occludens 1 PDZ1 (ZO-1-PDZ1) representing class III (D/E-X-Φ) ( Fig. 4a ) [20] . In addition, these PDZ domains also represent domains with fewer binding partners (nNOS-PDZ), as well as more promiscuous PDZ domains (ZO-1-PDZ1) [22] . We subjected the four PDZ domains to the same procedures employed for PSD-95-PDZ2. Suitable ligation sites were identified by Cys mutagenesis ( Supplementary Fig. 4 ), the applied EPL strategy ( Fig. 1c ) was verified by semisynthesis of WT SS PDZ domains, followed by assessment of the secondary structure ( Supplementary Fig. 5 ) and ligand-binding ( Fig. 4b ). Gratifyingly, all four PDZ domains were amenable to semisynthesis, and single A-to-E mutations were introduced into the carboxylate-binding site (Φ 1 , G and Φ 2 ) in each of the four PDZ domains (MPP7-PDZ: L149λ, G150γ, A151α; RGS3-PDZ: F28ϕ, G29γ, F30ϕ; nNOS-PDZ: L28λ, G29γ, F30ϕ; ZO-1-PDZ1: F34ϕ, G35γ, I36τ). 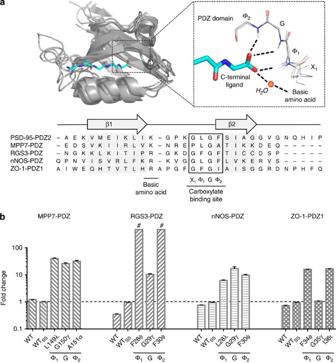Figure 4: Binding of C-terminal peptide ligands to backbone-modified PDZ domains. (a) X-ray crystal structures and sequence alignment of the included class I (PSD-95-PDZ2), II (MPP7-PDZ and RGS3-PDZ) and III (nNOS-PDZ and ZO-1-PDZ1) PDZ domains. The structure of a C-terminal ligand (light blue) and five PDZ domains (grey) show overlapping backbone at G and Φ2of the carboxylate-binding site, whereas the backbone structures of X1and Φ1are less preserved (PDB ID 3GSL, 1QAV, 3O46, 2F5Y and 2H2C). (b) Affinity fold change of class II and III semisynthetic PDZ domains from FP assay (calculated asKd(mutant)/Kd(WTSS)±s.e.m). The binding constants of two class II C-terminal peptides (IDESKKEWLI and MHIQEKGFHV) were determined towards MPP7-PDZ and RGS3-PDZ, respectively, whereas the binding constants for the class III peptide (HSGYRLDNDYV) were determined towards nNOS and ZO-1-PDZ1. The peptides were fluorescently labelled with TAMRA (SeeSupplementary Fig. 6for the affinity constants). # indicates >100-fold decrease in affinity. For the semisynthetic RGS3-PDZ domains, three point mutations were introduced (C73S, C83S, C112S) in the expressed fragment for semisynthetic feasibility, which only induced a modest change in affinity (Kd(WT)=1.8±0.1 μM andKd(WTSS)=5.0±0.1 μM). Figure 4: Binding of C-terminal peptide ligands to backbone-modified PDZ domains. ( a ) X-ray crystal structures and sequence alignment of the included class I (PSD-95-PDZ2), II (MPP7-PDZ and RGS3-PDZ) and III (nNOS-PDZ and ZO-1-PDZ1) PDZ domains. The structure of a C-terminal ligand (light blue) and five PDZ domains (grey) show overlapping backbone at G and Φ 2 of the carboxylate-binding site, whereas the backbone structures of X 1 and Φ 1 are less preserved (PDB ID 3GSL, 1QAV, 3O46, 2F5Y and 2H2C). ( b ) Affinity fold change of class II and III semisynthetic PDZ domains from FP assay (calculated as K d (mutant)/ K d (WT SS )±s.e.m). The binding constants of two class II C-terminal peptides (IDESKKEWLI and MHIQEKGFHV) were determined towards MPP7-PDZ and RGS3-PDZ, respectively, whereas the binding constants for the class III peptide (HSGYRLDNDYV) were determined towards nNOS and ZO-1-PDZ1. The peptides were fluorescently labelled with TAMRA (See Supplementary Fig. 6 for the affinity constants). # indicates >100-fold decrease in affinity. For the semisynthetic RGS3-PDZ domains, three point mutations were introduced (C73S, C83S, C112S) in the expressed fragment for semisynthetic feasibility, which only induced a modest change in affinity ( K d (WT)=1.8±0.1 μM and K d (WT SS )=5.0±0.1 μM). Full size image The resulting 16 semisynthetic PDZ domains were refolded and examined by CD analysis ( Supplementary Fig. 5 ) and their ligand-binding properties were determined in FP assays ( Supplementary Fig. 6 ). All proteins displayed similar overall curvature as the WT and WT SS proteins, indicating that all A-to-E-mutated PDZ domains were folded. For the class II PDZ domains MPP7-PDZ and RGS3-PDZ, a substantial decrease in affinity was observed by the A-to-E mutations ( Fig. 4b ). The F28ϕ and F30ϕ mutations in RGS3-PDZ displayed the most pronounced decreases in affinity with estimated K d values of >700 μM and >1,000 μM, respectively, corresponding to >100-fold loss of affinity. In contrast, the G29γ mutation was much less affected (11-fold loss in affinity). The corresponding mutations in MPP7 caused a 40-, 26- and 31-fold loss in affinity for L149λ, G150γ and A151α, respectively. The class III PDZ domains nNOS-PDZ and ZO-1-PDZ were generally less affected by the A-to-E mutations. The mutations in nNOS-PDZ caused a 7-, 19- and 11-fold loss of affinity for the peptide ligand for L28λ, G29γ and F30ϕ mutations, respectively, while the binding affinities to ZO-1-PDZ were reduced 18- and 19-fold for F34ϕ and I36τ mutations, respectively; however, the G35γ mutation did not cause a change in binding affinity. The ZO-1-PDZ1 domain has at least 22 known endogenous C-terminal peptide-binding partners [22] , and here we employed the class III sequence (HSGYRLDNDYV) as ligand. We also examined the binding affinity for another endogenous C-terminal ligand (PSIYSKSQYV) to the same ZO-1-PDZ1 A-to-E mutants, showing similar fold changes in ligand affinity to those found for HSGYRLDNDYV ( Supplementary Fig. 7 ). This demonstrates that changes in P -2 of the ligand (D versus Q) do not affect the H-bond pattern between the peptide ligand and the carboxylate-binding site. These results also show that different peptide ligands share similar H-bond patterns for a given PDZ domain. Backbone H-bonds in non-canonical β-finger interactions The interactions of nNOS with PSD-95, syntrophin and ZO-1 (ref. 28 ) are mediated via a non-canonical interaction, where an internal β-finger motif of nNOS is accommodated in the peptide-binding groove of the PDZ domain [26] . Although there is no C-terminal carboxylate involved in ligand binding, structural studies suggest that at least three backbone H-bonds from backbone amides of the PDZ domain are formed [26] ( Fig. 1b ). In general, only very few functional studies of β-finger interaction to the PDZ domains have been performed [27] , [47] , [48] . Thus, to investigate the role of the H-bonds in this non-canonical interaction we evaluated our A-to-E mutants of PSD-95-PDZ2 and ZO-1-PDZ1 for binding to the β-finger motif of nNOS. First, we prepared a fluorescent mimic of the nNOS β-finger as the full-length nNOS is not suitable as ligand in the FP assay. The cyclic [49] 5/6-tetramethylrhodamine (TAMRA)-labelled β-finger mimic 5 was generated by backbone cyclization via native chemical ligation ( Fig. 5a ) and subsequent attachment of a TAMRA fluorophore. The binding affinities of 5 to WT ( K d =1.2±0.11 μM) and WT SS PSD-95-PDZ2 ( K d =1.8±0.0095 μM) ( Supplementary Fig. 8 ) were similar to the K d value for nNOS/PSD-95 interaction previously reported ( K d =1 μM) [27] , [48] verifying that the β-finger mimic 5 can be used to examine the binding mode of full-length nNOS. We then determined the binding affinities of 5 for the five PSD-95-PDZ2 A-to-E mutants ( Fig. 5b and Supplementary Fig. 8 ). In general, binding of the β-finger ligand is much less affected by the A-to-E mutations compared with the linear C-terminal peptide ligand ( Fig. 3a ). A-to-E mutations in the carboxylate-binding site and the G176 position caused less than sevenfold change in affinity towards the β-finger 5 , which reinforces that A-to-E mutations can be introduced in the carboxylate-binding site without perturbing the backbone structure of this loop. In contrast, the I174τ mutation in the β2 strand leads to a major reduction in affinity (89-fold). Thus, these results suggest that the binding mode of the β-finger ligand of nNOS to PSD-95-PDZ2 is noticeably different from that of the linear C-terminal peptide. 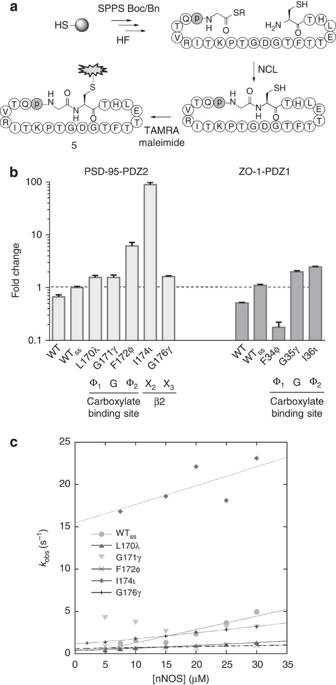Figure 5: Non-canonical ligand binding to A-to-E-mutated PDZ domains. (a) Synthesis of a fluorescent probe for investigating non-canonical β-finger/PDZ domain interaction in the FP assay. A peptide sequence resembling a modified β-finger from nNOS was synthesized using Boc/Bn-based SPPS, cleaved with HF and backbone-cyclized via native chemical ligation (NCL). The peptide was subsequently reacted with TAMRA-maleimide generating the β-finger probe5. (b) Affinity fold change for the β-finger mimic5and the semisynthetic A-to-E mutants of PSD-95-PDZ2 and ZO-1-PDZ (Kd(mutant)/Kd(WTSS)±s.e.m) (SeeSupplementary Fig. 8for the affinity constants). (c) Observed rate constants (kobs) for the binding of PSD-95-PDZ2 (WTSSand A-to-E mutants) to the β-finger of nNOS-PDZ. Figure 5: Non-canonical ligand binding to A-to-E-mutated PDZ domains. ( a ) Synthesis of a fluorescent probe for investigating non-canonical β-finger/PDZ domain interaction in the FP assay. A peptide sequence resembling a modified β-finger from nNOS was synthesized using Boc/Bn-based SPPS, cleaved with HF and backbone-cyclized via native chemical ligation (NCL). The peptide was subsequently reacted with TAMRA-maleimide generating the β-finger probe 5 . ( b ) Affinity fold change for the β-finger mimic 5 and the semisynthetic A-to-E mutants of PSD-95-PDZ2 and ZO-1-PDZ ( K d (mutant)/ K d (WT SS )±s.e.m) (See Supplementary Fig. 8 for the affinity constants). ( c ) Observed rate constants ( k obs ) for the binding of PSD-95-PDZ2 (WT SS and A-to-E mutants) to the β-finger of nNOS-PDZ. Full size image We next examined the binding of 5 to WT and A-to-E mutants of ZO-1-PDZ1. K d values for binding of 5 to WT and WT SS ZO-1-PDZ1 ( Fig. 5b ) were comparable to the nNOS/ZO-1-PDZ1 interaction [28] . The binding of 5 to the three ZO-1-PDZ1 A-to-E mutants showed only very modest decreases in affinity for the G35γ and I36τ mutants ( Fig. 5b ), whereas the F34ϕ mutation caused a 13-fold increase in affinity. Together, these results demonstrate that the C-terminal peptide and β-finger ligands bind in two distinct modes with different H-bond patterns to PDZ domains. The relatively small change in affinity for the β-finger ligand binding produced by the A-to-E mutants of PSD-95-PDZ2 was confirmed by kinetic stopped-flow experiments. Binding reactions of WT and A-to-E mutants of PSD-95-PDZ2 to the nNOS β-finger were measured to obtain k on and k off values ( Fig. 5c and Supplementary Table 2 ) [48] . Interestingly, the binding kinetics between L170λ and F172ϕ mutants and the nNOS β-finger were very different from those of the C-terminal ligand. The k on values for binding of nNOS β-finger to L170λ and F172ϕ mutants of PSD-95-PDZ2 decreased 4- and 12-fold, respectively ( Fig. 5c , Supplementary Table 2 ). This suggests that these backbone amides are important during the association of PSD-95-PDZ2 and the nNOS β-finger. However, since these mutations also resulted in reduced k off values, the H-bond interactions may be non-favourable or not relevant in the bound complex. For the G171γ mutation, the k on was found to be independent of the concentration of nNOS β-finger. The k off of G171γ (4.1 s −1 ) and the K d value suggest that the G171γ mutation has changed the binding reaction mechanism to include a slow conformational change before the association with the β-finger. Thus, the kinetics of all three A-to-E mutants suggests an important mechanistic role of the backbone amide NH for the early events of the binding reaction, perhaps transient formation of H-bonds. However, it is clear that the H-bonds do not contribute to the affinity of the bound complex. Finally, the I174τ mutation was not found to affect k on . Therefore, the destabilization ( ca . 1.2 kcal mol −1 ) of the bound complex observed by this mutation is entirely caused by changes in k off , suggesting that this backbone amide makes a H-bond to the β-finger of nNOS in agreement with the FP data and the X-ray crystal structure of syntrophin-PDZ with the PDZ domain of nNOS where the β-finger is situated [26] . In the current study, we have addressed key aspects of the molecular mechanisms and determinants underlying ligand/PDZ domain interactions. Specifically, we have examined the contribution of H-bond interactions of backbone amide NH groups in and near the carboxylate-binding site in PDZ domains for the canonical interaction of the carboxylate group of C-terminal peptide ligands, as well as for the non-canonical β-finger interaction. Although the importance of the carboxylate-binding site has long been acknowledged, very few studies have addressed the role of the backbone H-bonds that are assumed to be major contributors of the interaction between the C-terminal peptide ligand and the carboxylate-binding site ( Fig. 1a ) [45] , [46] . A major reason for this lack of studies is likely the methodological challenges of addressing backbone interactions in general. However, semisynthetic strategies for generation of proteins comprising backbone modifications such as the A-to-E mutation can be used to site-specifically address backbone H-bond interactions without perturbing the overall structure of the protein. In this study, we set out to establish a semisynthetic method to generate PDZ domains to enable introduction of A-to-E mutations in the carboxylate-binding site, as well as other relevant sites in the β2 strand of prototypical PDZ domains. This was achieved by a combination of SPPS and recombinant protein expression, and the feasibility of the developed semisynthetic strategy was demonstrated by generation of 22 semisynthetic PDZ domains, whereof 17 contained A-to-E mutations, in sufficient quantities for ligand-binding studies. Notably, the versatility of our methodology also allows the introduction of a much wider range of modifications such as biophysical probes and site-specific post-translational modifications, which are known to play important roles in regulation of PDZ domain function [4] , [6] . The binding profiles of five A-to-E mutants of PSD-95-PDZ2 provide several new insights into the molecular determinants for PPI interactions mediated by PDZ domains. Structural studies have suggested a number of H-bond interactions from the carboxylate-binding site and the β2 strand; however, the individual importance of these has not been addressed. Here we find that a single amide NH interaction in the β2 strand (I174) and three amide NH in the carboxylate-binding site contribute to the binding affinity in PSD-95-PDZ2. In the generally accepted binding mode ( Fig. 1a ), the amide NH of G176 located in the β2 strand is oriented towards the carbonyl amide of the peptide ligand backbone (P -4 residue). However, an A-to-E mutation in this position does not affect binding affinity, suggesting that a H-bond is not formed. The backbone amide at I174, also located in the β2 strand, forms a H-bond to the carbonyl of P -2 in the peptide ligand and A-to-E mutation produces a 50-fold loss of affinity. This suggests an essential role in ligand/PDZ interaction for this backbone amide NH, equally important as coordinating the carboxylate-binding site. In current models for ligand binding to PDZ domains, the relative contributions by the amide NH in the carboxylate-binding site are unknown; however, here we show that removal of the NH-mediated H-bond of G171 in PSD-95-PDZ2 does not affect the affinity to the same extent as for L170 and F172 ( Fig. 3b ). The changes in binding energy induced by the protein A-to-E mutations correlate well with our recent study, where backbone mutations of peptide ligands were used to elucidate the role of backbone H-bonds [46] . It was found that interactions from the backbone amides in positions P 0,-1 , P -1,-2 and P -2,-3 of the peptide ligand contributes exclusively to binding (ΔΔ G >1.3 kcal mol −1 ) in contrast to the amide at P -3,-4 (ΔΔ G =0.15 kcal mol −1 , Fig. 6a and Supplementary Table 3 ) [46] . These observations support the findings from the present study, where the change in binding energy for the protein A-to-E mutations of the I174 and G176 is determined to ΔΔ G =2.1 kcal mol −1 and ΔΔ G =0.16 kcal mol −1 , respectively ( Supplementary Table 3 ). 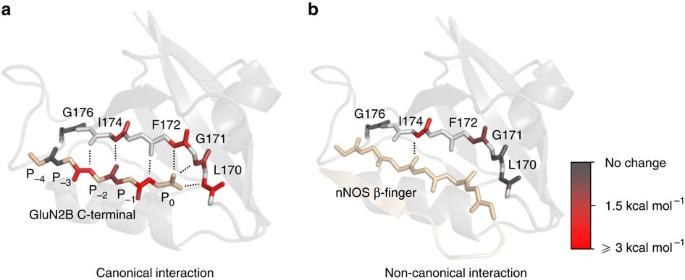Figure 6: H-bonding energy contributions for PSD-95-PDZ2 studied by A-to-E mutations. (a) H-bond contribution for the canonical interaction between GluN2B peptide46(light brown) and PSD-95-PDZ2 domain (light grey). Six H-bonds (dotted lines) were found to significantly contribute to the affinity of the interaction (ΔΔGmutant–WT>1.3 kcal mol−1) extending from the carboxylate-binding site to I174/P-2,-3, whereas the amide NH of G176 and carbonyl of P-3,-4are not implicated in H-bond formation in the canonical binding mode. (b) H-bond contributions in the non-canonical interaction between nNOS β-finger (brown) and PSD-95-PDZ2 (light grey). One of the five tested H-bonds, amide NH from I174 (ΔΔG=2.5 kcal mol−1), contributes to the binding energy during equilibrium. However, the association rate constants for all A-to-E mutations except I174τ are decreased (Supplementary Table 2,Fig. 5c), demonstrating that these amide NH groups play a role during the binding reaction, possibly by forming transient H-bonds. Protein structures are models adapted from PSD-95-PDZ3/CRIPT (PDB ID 1BE9) and syntrophin-PDZ/nNOS-PDZ (PDB ID 1QAV). SeeSupplementary Table 3for actual values. Figure 6: H-bonding energy contributions for PSD-95-PDZ2 studied by A-to-E mutations. ( a ) H-bond contribution for the canonical interaction between GluN2B peptide [46] (light brown) and PSD-95-PDZ2 domain (light grey). Six H-bonds (dotted lines) were found to significantly contribute to the affinity of the interaction (ΔΔ G mutant–WT >1.3 kcal mol −1 ) extending from the carboxylate-binding site to I174/P -2,-3 , whereas the amide NH of G176 and carbonyl of P -3,-4 are not implicated in H-bond formation in the canonical binding mode. ( b ) H-bond contributions in the non-canonical interaction between nNOS β-finger (brown) and PSD-95-PDZ2 (light grey). One of the five tested H-bonds, amide NH from I174 (ΔΔ G =2.5 kcal mol −1 ), contributes to the binding energy during equilibrium. However, the association rate constants for all A-to-E mutations except I174τ are decreased ( Supplementary Table 2 , Fig. 5c ), demonstrating that these amide NH groups play a role during the binding reaction, possibly by forming transient H-bonds. Protein structures are models adapted from PSD-95-PDZ3/CRIPT (PDB ID 1BE9) and syntrophin-PDZ/nNOS-PDZ (PDB ID 1QAV). See Supplementary Table 3 for actual values. Full size image To investigate the generality of the H-bonding pattern in the canonical ligand binding to other classes of PDZ domains, we examined four additional PDZ domains in a similar manner. Alignment of X-ray crystal structures of PDZ domains shows a high degree of structural conservation among G-Φ 2 residues, whereas the X 1 -Φ 1 residues show more flexibility ( Fig. 4a ). For three of the four PDZ domains, we observe a very similar pattern, in which the amide of the conserved G residue is relatively less important for ligand binding, compared with the two neighbouring amides, Φ 1 and Φ 2 ( Fig. 4b ). Both NH groups of Φ 1 and Φ 2 are directed towards the carboxylate group and stabilize the carboxylate from both sides [18] . Thus, removing the amides by A-to-E mutations disrupts the coordination of the carboxylate, and the peptide interaction is significantly weakened. The orientation of the backbone amide NH from G is different due to a conserved left-handed α-helical turn in the backbone ( Fig. 4a ), which is unfavourable for H-bond formation ( Supplementary Table 4 ). This is supported in our studies, where we observed a relatively lower fold change upon A-to-E mutation of the G position. A notable exception is seen in nNOS-PDZ, where A-to-E mutation of G (G35γ) leads to the largest loss of ligand affinity, which could indicate that the coordination of the C-terminal carboxylate in nNOS-PDZ is different from the interaction in the four other PDZ domains. Since structural studies have suggested similar backbone structures and orientation of the backbone amide NH towards the carboxylate ( Fig. 1a ), it is surprising that we find very pronounced differences in the effects on ligand affinity of A-to-E mutations across the five PDZ domains. One possible explanation is that the C-terminal carboxylate of the ligand positions differently towards the carboxylate-binding site of the PDZ domains and thereby attains subtle differences in H-bond patterns, which also has been suggested by X-ray crystal structures of PDZ domains in complex with C-terminal ligands [50] . These findings together with our present data suggest that the C-terminal interaction at the carboxylate-binding site could be part of a selectivity mechanism that allows the PDZ domains to discriminate between C-terminal peptide ligands [51] . We also examined the non-canonical interaction of a β-finger ligand, as found in nNOS β-finger binding to PSD-95 and syntrophin [26] , [27] , [47] . For this interaction, we observe a striking and fundamental difference from the canonical interaction. An X-ray crystal structure of a β-finger/PDZ domain interaction displays backbone H-bond interactions similar to those of the canonical C-terminal peptide [26] ( Fig. 1a,b ). Our findings show that A-to-E mutations of Φ 1 (L170λ in PSD-95-PDZ2 and F34ϕ in ZO-1-PDZ1) do not negatively affect β-finger ligand-binding ( Fig. 5b ), consistent with X-ray crystallographic data. For putative H-bonds from backbone NH of Φ 2 and G, the A-to-E mutations show noticeable differences in binding to C-terminal peptide or β-finger ligand. For mutations in both PSD-95-PDZ2 (G171γ and F172ϕ) and ZO-1-PDZ1 (G35γ and I136τ), the affinity of the β-finger ligand is not perturbed ( Fig. 5b ), thus disagreeing with H-bond interactions suggested by structural studies [26] . In contrast, we find that establishing the H-bond from X 2 in the β2 strand is by far the most important H-bond for the non-canonical β-finger interaction. Specifically, we observed that the X 2 mutation (I174τ) in PSD-95-PDZ2 causes a 90-fold reduction in ligand-binding affinity for the β-finger interaction, whereas none of the other A-to-E mutations causes >10-fold change in affinity ( Figs 3b and 5b ). Finally, G176 in PSD-95-PDZ2 does not seem to be important for non-canonical ligand binding ( Fig. 5b ), thereby indicating that the NH of X 3 in the β2 strand is not forming an H-bond to the ligand similarly to what was observed for the canonical interaction ( Fig. 3a ). In summary, our results demonstrate striking and unanticipated differences between the two predominant modes of ligand/PDZ domain interactions ( Fig. 6 ). These results provide detailed insight into the relative importance of H-bonds for PDZ/ligand interactions, which is important for understanding fundamental aspects of this class of scaffolding proteins. Future studies such as X-ray crystal structures of PDZ domains with A-to-E mutations could provide additional and seminal information on these interactions. PDZ domains are also emerging as feasible and highly attractive drug targets, particularly in the development of neuroprotective agents targeting PSD-95, such as the treatment of ischemia, pain and depression [10] , [11] , [12] , [13] , [14] . The most promising lead structures are all peptide-based, and development of potent small molecule inhibitors of PDZ domains has proven challenging [10] . However, the current study now provides an improved frame for developing new and better inhibitors, allowing a rational approach for developing ligands that exploit the key H-bonds for PDZ/ligand interactions found here. In conclusion, we have developed a general methodology for the semisynthesis of PDZ domains, and have exploited this for elucidating the functional importance of H-bonding in the ligand-binding site of PDZ domains. We hereby enable specific quantification of the contributions of individual backbone amide NH to ligand binding in PDZ domains, which provides novel insights into the overall role of backbone interactions and reveals important differences among PDZ domains in their recognition of canonical and non-canonical ligands. Moreover, these findings contribute a new aspect to the molecular mechanism underlying ligand selectivity of PDZ domains, which so far is not fully understood. Our results expand the structural framework concerning PDZ domain interactions that can be benefitted to explore development of PDZ inhibitors to dissect the physiological role of PDZ domains or as putative drugs targeting specific PDZ domains. Peptide synthesis Unless otherwise stated, starting materials were obtained from commercial suppliers and used without further purification. Boc- and Fmoc-protected AA, coupling reagents and trifluoroacetic acid (TFA) were purchased either from Peptides International (Louisville, KY, USA) or Iris Biotech (Marktredwitz, Germany). 4-benzyloxybenzyl alcohol (Wang) resins were purchased containing a Fmoc-protected Val, Ile or Phe from Iris Biotech, preloaded trityl- S -mercaptopropionic Leu 4-hydroxymethyl-phenylacetamidomethyl (PAM) resin from Peptides International and 2-(3,5-dimethoxy-4-formylphenoxy)ethyl polystyrene resin from Merck (Whitehouse Station, NJ, USA). Peptide synthesis was performed in 0.25 mmol scale and carried out manually or using an automated microwave peptide synthesizer with a Discover microwave reactor connected to a Liberty module (CEM Corporation, Matthews, NC, USA). For each programmed coupling cycle, Fmoc-based coupling was achieved with 4 equiv. Fmoc-AA-OH, 4 equiv. 2-(1-benzotriazole-1-yl)-1,1,3,3-tetramethyluronium hexafluoro-phosphate (HBTU) and 4 equiv. N , N -diisopropylethylamine (DIPEA); Boc-based couplings were achieved with 4:4:8 (Boc-AA-OH:HBTU:DIPEA). Microwave coupling proceeded for 5 min (23 W, 75 °C). Fmoc deprotections were carried out with 20% piperidine in dimethylformamide (DMF) using microwave heating for 3 min (35 W, 75 °C). Boc deprotections were carried out with neat TFA for 1 min. Fmoc-based peptides were cleaved from the Wang resin with a mixture of TFA/water/triisopropylsilane (9:0.5:0.5) for 1 h, followed by removal of TFA and precipitation of the peptide with ice-cold diethyl ether. Boc-based peptides were cleaved from the PAM resin using hydrogen fluoride (HF)-reaction apparatus (Peptide International). The peptides were treated with anhydrous HF/p-cresol (9:1) for 1 h at 0 °C unless they contained His(benzyloxymethyl) in which a scavenger mix of anhydrous HF/p-cresol/resorcinol (9:0.5:0.5) was used. After HF evaporation, the peptide was precipitated with cold diethyl ether. The precipitate was dissolved in 20% aqueous MeCN containing 1% TFA. Peptides were purified by preparative reverse phase high-performance liquid chromatography (RP-HPLC) using a Agilent 1200 system with a C18 reverse phase column (Zorbax 300 SB-C18, 21.2 mm × 250 mm) with a linear gradient using binary solvent systems, H 2 O/MeCN/TFA (A: 95/5/0.1; B: 5/95/0.1). Mass spectra were obtained with an Agilent 6410 Triple Quadrupole Mass Spectrometer instrument using electron spray ionization (ESI) coupled to an Agilent 1200 HPLC system (ESI-LC/MS) with a C18 reverse phase column (Zorbax Eclipse XBD-C18, 4.6 mm × 50 mm), auto sampler and diode array detector using a linear gradient of the binary solvent system of H 2 O/MeCN/formic acid (A: 95/5/0.1; B: 5/95/0.086) with a flow rate of 1 ml min −1 . During ESI-LC/MS analysis, evaporative light scattering traces were obtained with a Sedere Sedex 85 Light Scattering Detector. The purities were estimated using analytical HPLC performed on an Agilent 1100 system with a C18 reverse phase column (Zorbax 300 SB-C18 column, 4.6 mm × 150 mm), flow rate of 1 ml min −1 and a linear gradient of the binary solvent system of H 2 O/MeCN/TFA (A: 95/5/0.1; B: 5/95/0.1). The final products were lyophilized ( Supplementary Table 5 ). α-Hydroxy acids were either purchased (Sigma-Aldrich) or synthesized using a modified diazotization protocol from Deechongkit and Kelly [41] . Incorporation into peptide sequence was performed according to a protocol described by Beligere and Dawson [40] . Fluorescent peptides were synthesized using Fmoc-based SPPS having a TAMRA at the N-terminal. The fluorophore was coupled on resin using a mixture of TAMRA/HBTU/DIPEA (4:4:4) dissolved in DMF/DCM (1:1, 2 ml) for 15 min. Cy5 maleimide (Anaspec) was coupled on an N-terminal cysteine in solution after initial purification. Peptide (2 mg, 1.31 mmol) was mixed with Cy5 maleimide (1 mg, 1.22 mmol) and dissolved in phosphate-buffered saline (2 ml). The coupling was carried out at room temperature for 2 h. The crude peptides were purified with RP-HPLC, monitoring at λ 470nm /λ 544 nm and subsequently characterized by LC-MS ( Supplementary Table 5 ). The cyclic peptide probe was prepared by Boc-based SPPS inspired by work of Seedorf et al. [49] A linear peptide was synthesized on a preloaded trityl- S -mercaptopropionic Leu PAM resin having an N-terminal L -thiazolidine and a D -proline (p). After HF cleavage (15 ml, 1 h, 0 °C), the peptide was dissolved in buffer (0.3 M methoxyamine, 0.1 M acetate, pH 4, 200 ml), purified by preparative RP-HPLC and lyophilized. The cyclic peptide was dissolved in phosphate-buffered saline buffer (2 ml), and 5-TAMRA C2 maleimide (1 mg, Anaspec) was added and incubated for 2 h at 37 °C. The product was purified by preparative RP-HPLC, monitoring at λ 554 nm and characterized by LC-MS ( Supplementary Table 5 ). Vector design and expression The expression vector pRSET was purchased from Invitrogen (Carlsbad, CA, USA). Codon-optimized DNA constructs containing PDZ domains were purchased from Invitrogen containing HindIII and KpnI surrounding the PDZ insert. All constructs were verified by DNA sequencing (Eurofins MWG Operon, Germany). The pRSET vector was amplified by polymerase chain reaction (Quickchange kit, Stratagene, CA, USA) using the primers encoding HindIII restricting sites aspRSET-HindIII (5′-CGCCCGGAATATGCTGGTTAAGCTTACGGCCTTCAATGCCGCCGTG-3′) upstream the polyhistidine (7 × His) tag and KpnI site spRSET-KpnI (5′-CTGAAAGTGGCGAAACCGAGCGGTACCTAATAATAGCTTGATCCGGCTGCTAAC-3′) in front of the stop codon within the open reading frame. The product was digested with HindIII and KpnI along with the purchased PDZ inserts and the two fragments were ligated together using Roche Rapid DNA ligation Kit (Roche, Penzberg, Germany). The cysteine mutations were introduced by standard site-directed mutagenesis protocol (Stratagene). Following mutations were prepared: PSD-95-PDZ2: V178C, N180C, Q181C, H182C; MPP7: D256C; nNOS-PDZ: V36C; and ZO-1-PDZ1: R42C. The FXa sites were introduced by polymerase chain reaction amplification with elongated (+16 bp) primers sFXA (5′-NNNATCGAGGGAAGGTGTNNN-3′) and asFXA, thereby inserting four extra AA (Ile-Glu-Gly-Arg) next to the cysteine mutation. The mutations were introduced in PSD-95-PDZ2, MPP7-PDZ, RGS3-PDZ, nNOS-PDZ and ZO-1-PDZ1. Futhermore, three cysteines (C73, C83 and C112) of RGS-PDZ were mutated into serines by site-directed mutagenesis for semisynthetic feasibility. E. coli BL21 competent cells (DE3, pLysS, Stratagene) were transformed with plasmid containing WT or modified PDZ domains and grown on ampicillin-containing plates (100 μg ml −1 ) overnight (ON) at 37 °C. Colonies were used to inoculate 10-ml preculture (100 μg ml −1 ampicillin) lysogeny broth medium (10% tryptone, 5% yeast extract, 10% NaCl and 0.8% glucose, pH 7.2) which was left in a rotary shaker ON at 37 °C (240 r.p.m.). Growth flasks (2.5 l) were autoclaved with 1 l auto-induction medium ZYM5052. The medium was preheated to 37 °C and prepared with ampicillin (50 μg ml −1 ). The ON culture was poured into the ZYM medium and incubated in a rotary shaker (37 °C, 210 r.p.m.). The cell density was monitored by optic density at 600 nm on a 96-well plate (transparent, flat-bottom, Corning Life Science, NY, USA) using a Safire plate-reader (Tecan, Männendorf, Switzerland). After reaching optic density ~0.6, the temperature was reduced to 30 °C and the cells were left ON. Cells were harvested by centrifugation (10,000 × g , 15 min) and resuspended in 50 ml lysis buffer (50 mM Tris-HCl, 1 mM phenylmethanesulfonylfluoride (Sigma-Aldrich), 25 μg ml −1 Dnase (Sigma-Aldrich), 40 mg ml −1 MgSO 4 ). The suspension was processed in a cell-disrupter apparatus (Constant Systems Ltd, Darventry, England) at 26 kPsi and collected in falcon tubes containing solid GuHCl, giving a final concentration of ~6 M. The mixture was incubated at 37 °C at 240 r.p.m. for 30 min and afterwards spun down at 50,000 × g for 1 h. The supernatant was adjusted with 2 M NaOH to a pH of ~7.5. An ÄKTA Explorer 100 Air (GE Healthcare Life Sciences, Uppsala, Sweden) system was used for purifying the proteins on 2 × 5 ml HisTraps (GE Healthcare Life Sciences) loaded with Ni 2+ -charged resin material that was equilibrated with wash buffer (6 M GuHCl, 300 mM NaCl, 50 mM NaPi, 25 mM imidazole, pH 7.5). The cell lysate was loaded on the HisTraps (1 ml min −1 ) by a 50 ml SuperLoop (GE Healthcare Life Sciences). Twenty-five milliliter wash buffer (2 ml min −1 ) was used to remove impurities followed by a gradient elution (0–100% over 25 min, 1 ml min −1 ) with elution buffer (6 M GuHCl, 300 mM NaCl, 50 mM NaPi, 250 mM imidazole, pH 8.0). The elution was monitored at λ 280 and the eluate was collected in 5-ml aliquots, which were subsequently analysed using SDS–polyacrylamide gel electrophoresis and pooled. The N-terminal Cys fragments were expressed and subjected to Ni 2+ -based purification as described for the full-length PDZ domains. After Ni 2+ -based purification, the purified protein stocks were subsequently dialysed in SnakeTubes (Sigma-Aldrich) with a molecular cutoff at 7 kD into FXa-buffer (20 mM Tris, 50 mM NaCl, 1 mM CaCl 2 ) three times at 4 °C, the last time being ON. Any precipitated protein was removed with centrifugation (3,500 × g , 15 min). FXa enzyme (Qiagen, Hilden, Germany) was added to a final concentration of 2 units ml −1 and incubated 24 h at 4 °C. Solid GuHCl, NaCl and imidazole were added to the protein solution giving a final concentration of 4 M, 300 mM and 25 mM, respectively, and pH was adjusted to pH 7.5 after mixing. The N-terminal Cys protein was repurified using HisTraps where the truncated protein was collected in the flow-through. The flow-through was desalted by dialysis in SnakeTube (Sigma-Aldrich) into water. The dialysate was lyophilized forming a white amorphous product, which was characterized by analytical HPLC and LC/MS ( Supplementary Table 6 ). Ligation and refolding All ligations were initiated by dissolving the ~5-mg lyophilized, expressed protein in 200 μl ligation buffer (200 mM NaPi, 6 M GuHCl, 30 mM mercaptophenyl acetic acid, 20 mM TRIS, TCEP, pH 7.1) in an Eppendorf tube. The lyophilized peptide was added afterwards. The product formation was monitored using LC/MS over 2 h. The reaction was stopped by adding 100 μl 1 M DTT followed by 5 ml 20% aqueous MeCN with 1% TFA. The ligation mixture was purified using RP-HPLC, lyophilized and characterized ( Supplementary Table 6 ). To ensure stability (avoid hydrolysis), the refolding of the A-to-E-mutated proteins was performed at pH 7.0 (instead of pH 7.4) and assays were conducted the same day. The lyophilized semisynthetic proteins were dissolved in a 100- to 400-μl denaturing buffer (6 M GuHCl, 0.1 M sodium acetate, pH 4), and 100 μl was transferred into soaked dialysis tubes (Pur-A-Lyzer Mini, Cutoff 6000, Sigma-Aldrich). The tubes were dialyzed in 1 l FP buffer (4 °C, 4 h). The concentration was determined using absorbance at λ 280nm measured on a NanoDrop 1000 spectrometer (Thermo Fisher Scientific, Waltham, MA, USA). Circular dichroism CD experiments were conducted on an Olis DSM 100 CD Spectrometer (Olis Inc, Bogart, GA, USA) in 1-mm quartz cuvettes (Starna Scientific Ltd, Essex, England). The CD spectrum was measured on protein samples with a concentration of ~10 μM, and the data were obtained in millidegrees of ellipticity, which was converted into mean residue ellipticity. Kinetic measurements Kinetic binding rate constants of PSD-95-PDZ2 were measured on an upgraded SX17 stopped-flow spectrometer from Applied Photophysics (Leatherhead, UK). The experiments were conducted at 10 °C in 50 mM potassium phosphate, 400 mM NaSO 4 , pH 7.0. Binding kinetics was measured either using a dansylated GluN2B C-terminal peptide, SIESDV or the the PDZ domain of nNOS containing the β-finger [48] . Excitation was at λ 280 nm and the change in Trp emission with time was recorded either above λ 320 nm using a cutoff filter or around λ 330 nm using an interference emission filter. All experimental traces followed single exponential kinetics, and observed rate constants were plotted versus the concentration of C-terminal peptide or nNOS-PDZ and fitted to the following equation (1) to obtain the association rate constant k on and the dissociation rate constant k off . [Ligand] is the concentration of either the C-terminal peptide or the nNOS-PDZ. The k off value for WT SS was not well defined from this extrapolation and determined in a separate displacement experiment as previously described [48] . Fluorescence polarization The FP assay was generally performed as previously described [39] . In brief, binding affinities were measured using a Safire plate-reader (Tecan) in a flat-bottom black 396-well plate (Corning Life Science). The buffer was either 50 mM NaPi pH 7.0/7.4 or 50 mM KPi, 400 mM NaSO 4 pH 7.0 including bovine serum albumin. Five to eight measurements were made for each binding setup and repeated three times. The TAMRA or Cy5-containing probes were measured at excitation/emission wavelengths of λ 545 nm /λ 575 nm and λ 470 nm /λ 525 nm , respectively. The concentration of the fluorescent probe was 50 nM in all the FP experiments. The instrumental Z-factor was adjusted to obtain maximum signal and the G-factor calibrated from the blank and background wells to give an initial milli-polarization of 20. The obtained saturation curve was subtracted from the background and fitted to one-sided binding model. If the K d for the investigated interaction was high (>50 μM), the B max values were constrained to the same B max as the corresponding WT. Data analysis All modelling figures were prepared using PyMOL (DeLano Scientific, Palo Alto, CA, USA). Analysis of functional and folding data was performed using the Prism 5.0 software (GraphPad Inc., San Diego, CA, USA) or Kaleidagraph (Synergy Software, Reading, PA, USA). How to cite this article: Pedersen, S. W. et al. Probing backbone hydrogen bonding in PDZ/ligand interactions by protein amide-to-ester mutations. Nat. Commun. 5:3215 doi: 10.1038/ncomms4215 (2014).